Graphene nanoelectronic heterodyne sensor for rapid and sensitive vapour detection Nearly all existing nanoelectronic sensors are based on charge detection, where molecular binding changes the charge density of the sensor and leads to sensing signal. However, intrinsically slow dynamics of interface-trapped charges and defect-mediated charge-transfer processes significantly limit those sensors’ response to tens to hundreds of seconds, which has long been known as a bottleneck for studying the dynamics of molecule–nanomaterial interaction and for many applications requiring rapid and sensitive response. Here we report a fundamentally different sensing mechanism based on molecular dipole detection enabled by a pioneering graphene nanoelectronic heterodyne sensor. The dipole detection mechanism is confirmed by a plethora of experiments with vapour molecules of various dipole moments, particularly, with cis - and trans -isomers that have different polarities. Rapid (down to ~\n0.1 s) and sensitive (down to ~\n1 ppb) detection of a wide range of vapour analytes is achieved, representing orders of magnitude improvement over state-of-the-art nanoelectronics sensors. Nanoelectronic devices based on nanomaterials such as nanowires, carbon nanotubes, graphene and transition metal dichalcogenides offer extremely large surface-to-volume ratios, high carrier mobility, low power consumption and high compatibility for the integration with modern electronic technologies [1] , [2] , [3] , [4] . These distinct advantages are being explored for a variety of sensing applications in both liquid and gas phases [5] , [6] , [7] , [8] . In particular, chemical vapour sensing is uniquely positioned to elucidate the fundamental molecule–nanomaterial interaction and provide a test bed for evaluating nanoelectronic-sensing performance without interference from solvent background typically seen in liquid-based detection [9] , [10] . The current signal of a nanoelectronic sensor can in general be expressed as: where G is the conductance, determined by the charge density of the device, Q ; is the conductance fluctuation and is related to the modulation of the charge density, ; V is the direct current (DC) voltage and is the alternating current (AC) excitation. Exploration of different terms in equation (1) can lead to different sensing mechanisms, for example, the first three terms have been employed in DC sensing, impedance sensing and noise sensing, respectively. In contrast, the fourth term explores the heterodyne mixing signal between conductance modulation and AC excitation, and has unfortunately been ignored in electronic-sensing techniques owing mainly to the lack of gain in conventional two-terminal devices. However, as we report in this article, utilizing the heterodyne mixing current as the sensing signal in a high-frequency graphene mixer will not only open up a new possibility of probing the fundamental molecule–graphene interaction, but, surprisingly, enable a rapid and sensitive nanoelectronic vapour sensor that significantly outperforms the current state-of-the-art. Presently the most common sensing mechanisms for nanoelectronic sensors, such as chemiresistors and transistor-based sensors, rely on the detection of charges. Charge transfer between the adsorbed molecules and the nanomaterial changes the surface charge density, thus altering the Fermi energy and conductance of the sensors [5] , [6] , [7] , [8] , [11] , [12] . Sensing is achieved by monitoring the DC conductance change (first term in equation 1) as a result of molecule–sensor interaction. To date, semiconductor nanowires, carbon nanotubes, graphene and MoS 2 have been explored as DC nanoelectronic vapour sensors [12] , [13] , [14] , [15] , [16] , [17] , with sensitivity down to the ppb level. However, the biggest challenge for such DC nanoelectronic vapour sensors is their extremely slow sensing response and recovery, typically on the order of tens to hundreds of seconds [7] , [8] , [12] , [13] , [14] , [15] . AC impedance-sensing technique utilizing the second term in equation 1 has also been demonstrated in chemicapacitors [18] . A carbon nanotube network-based chemicapacitor exhibited a detection limit of 50 ppb for dimethylmethylphosphonate (DMMP) [19] . However, a large device footprint (millimetre scale) is necessary for accurate capacitance measurement, and the use of chemoselective polymers in those devices significantly slows down the response time to hundreds of seconds. More recently, the low frequency noise spectrum of a graphene transistor was also used for chemical vapour sensing [20] by exploiting the third term in equation 1. Selective gas sensing was achieved on a single pristine graphene transistor, but the device suffered severely from extremely poor sensitivity and slow response time (>100 s). Unfortunately, the slow response for all existing nanoelectronic vapour sensors arises intrinsically from slow dynamics of interface-trapped charges and slow defect-mediated charge-transfer processes [21] , [22] , [23] , [24] , [25] , and therefore, is difficult, if not impossible, to overcome within the current framework of available sensing mechanisms. As a result, device regeneration is achieved only through prolonged heating, current stimulation or ultraviolet radiation [8] , [12] , [13] , [14] , [20] , [26] , [27] . Recently, various chemoselective surface coatings have been used [17] , [19] , [28] to reduce the response and recovery time to only a few seconds. However, those coatings function only for a narrow set of vapour molecules and may possibly result in even slower response to other vapour molecules [28] . All these drawbacks not only preclude studying the rapid dynamics of molecule–nanomaterial interaction, but also significantly hinder the employment of nanoelectronic sensors in applications like gas chromatography (GC), which require detection capability for a broad range of vapour analytes with sub-second response time and ppb-level sensitivity. Here we report a dipole-detection-based graphene nanoelectronic heterodyne sensor by exploiting the fourth term in equation 1. Different from all existing nanoelectronic-sensing technologies, our approach utilizes a graphene field-effect-transistor (GrFET) as a high-frequency (>100 kHz) mixer [9] , [29] with surface-adsorbed molecules functioning as an oscillating gate ( Fig. 1a ). The oscillating molecular dipole (excited by AC-driving voltage) induces a conductance modulation on the graphene channel; this conductance fluctuation is frequency-mixed with the AC excitation, thus generating a heterodyne mixing current. Importantly, by using higher frequencies, the slow sensing response hindering the conventional nanoelectronic sensor can be overcome when the AC field switching outpaces the slow dynamics of interface states. Therefore, our prototype graphene sensor can achieve simultaneously rapid (down to ~\n0.1 s) and sensitive (down to ~\n1 ppb) detection of a wide range of analytes, representing orders of magnitude improvement in both response time and sensitivity over state-of-the-art nanoelectronic sensors. 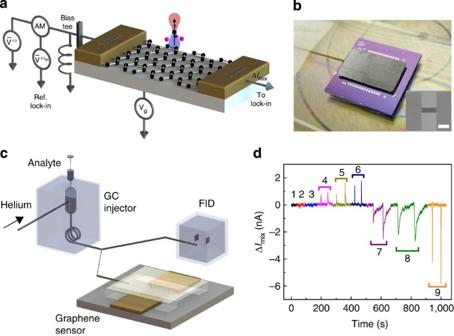Figure 1: Rapid and high-sensitivity graphene nanoelectronic heterodyne sensor. (a) Schematic showing a graphene transistor configured as a high-frequency mixer for heterodyne vapour sensing; and an illustration of a chloroform molecule on top of a graphene channel. The graphene sensor measures the mixing current between AC excitation and the dipole oscillation-induced charge density fluctuation. The arrow represents the dipole moment vector of chloroform. All vapour sensing were conducted atVsd=0 V,Vg=0 V, AC excitation frequencyω/2π=100 kHz, and AM modulation frequencyωm/2π=1.4342, kHz. (b) Optical image of the graphene sensor capped with a silicon flow channel and a GC guard column inserted at one end. The flow channel (dimensions—400 μm × 400 μm) was secured using a polymer adhesive at the edge. (Inset) scanning electron microscopy image of a typical graphene device. Scale bar, 5 μm. (c) Experimental setup showing a GC injector connected to the graphene sensor and a FID (a standard vapour detector with <0.1 s time resolution and <1 ppb sensitivity) through a GC separation column and a Y-split. (d) Mixing current response of a graphene heterodyne sensor to injections of various masses of (1) pentane, (2) hexane, (3) benzene, (4) chlorobenzene, (5) dichloromethane, (6) chloroform, (7) N, N-dimethylformamide (DMF), (8) DMMP and (9) acetone. Figure 1: Rapid and high-sensitivity graphene nanoelectronic heterodyne sensor. ( a ) Schematic showing a graphene transistor configured as a high-frequency mixer for heterodyne vapour sensing; and an illustration of a chloroform molecule on top of a graphene channel. The graphene sensor measures the mixing current between AC excitation and the dipole oscillation-induced charge density fluctuation. The arrow represents the dipole moment vector of chloroform. All vapour sensing were conducted at V sd =0 V, V g =0 V, AC excitation frequency ω/ 2 π =100 kHz, and AM modulation frequency ω m /2 π =1.4342, kHz. ( b ) Optical image of the graphene sensor capped with a silicon flow channel and a GC guard column inserted at one end. The flow channel (dimensions—400 μm × 400 μm) was secured using a polymer adhesive at the edge. (Inset) scanning electron microscopy image of a typical graphene device. Scale bar, 5 μm. ( c ) Experimental setup showing a GC injector connected to the graphene sensor and a FID (a standard vapour detector with <0.1 s time resolution and <1 ppb sensitivity) through a GC separation column and a Y-split. ( d ) Mixing current response of a graphene heterodyne sensor to injections of various masses of (1) pentane, (2) hexane, (3) benzene, (4) chlorobenzene, (5) dichloromethane, (6) chloroform, (7) N, N-dimethylformamide (DMF), (8) DMMP and (9) acetone. Full size image Graphene heterodyne vapour sensing setup Figure 1a illustrates the device design and working principle of our graphene nanoelectronic heterodyne sensor. An AC voltage at frequency ω , , is applied to the source electrode of a GrFET through a bias tee, while the DC bias at source and gate electrodes are held at ground ( V sd , V g =0 V). The electrostatic coupling between the graphene channel and the gate electrode leads to a gate-induced charge density modulation at ω , with C g being the gate capacitance per unit area and assuming perfect metal/graphene contacts. In the presence of a surface-adsorbed molecule, the oscillating molecular dipole can also lead to dipole-induced charge density modulation at ω , . The frequency mixing between and yields a heterodyne mixing current: where μ is the carrier mobility. W and L are the length and width of the device, respectively. For vapour sensing, the change in the mixing current is monitored as the sensing signal: For better noise rejection, an amplitude modulation on AC voltage drive can be applied, and the mixing current at the modulating frequency is detected using a lock-in amplifier (see Methods). To demonstrate vapour sensing, we fabricated GrFETs on silicon wafer with thermal oxide using chemical vapour deposition-grown graphene [30] , and integrated the graphene sensor with a standard GC system (see Methods and Supplementary Note 1 ). As shown in Fig. 1b , the GrFET die was capped with a 400-μm depth × 400-μm width-etched silicon-flow channel, before connecting to a 70-cm long GC guard column. The flow channel was carefully aligned to the centre of the die to ensure all the graphene sensors were exposed to the vapour flow. Analytes were injected using a syringe at the GC injection port, and delivered to the graphene sensor. Injected mass for each analytes was calibrated using a flame ionization detector (FID) ( Fig. 1c ). Fig. 1d shows the mixing current response of a typical graphene heterodyne sensor to nine different analytes including: (1) pentane, (2) hexane, (3) benzene, (4) chlorobenzene, (5) dichloromethane, (6) chloroform, (7) N , N -dimethylformamide, (8) DMMP and (9) acetone ( Supplementary Table 1 ). Rapid detections of six out of nine analytes were successfully demonstrated. Furthermore, initial results indicate that our graphene sensor was highly selective to polar molecules: three nonpolar molecules (pentane, hexane and benzene) showed no signal, while the remaining polar ones showed strong response. In addition, the sensing signal also appeared to have different signs for different molecules. Speed and sensitivity of graphene heterodyne vapour sensors Next, we investigated in detail the temporal response of the GrFET sensor to pulsed injections of varying masses of common volatile organic compounds. Some of the examples are shown in Fig. 2a . Significantly, fast sensor response with a sub-second full-width-half-maximum ( t 1/2 ) was observed for dichloromethane ( t 1/2 =0.61 s), ethanol ( t 1/2 =0.92 s), chloroform ( t 1/2 =0.69 s), 2-propanol ( t 1/2 =0.98 s) and acetone ( t 1/2 =0.75 s), which were similar to FID response times. Even for relatively high boiling point vapours—chlorobenzene, dioxane and N , N -dimethylformamide, whose boiling point is over 100 °C ( Supplementary Table 1 ), our graphene heterodyne sensors still showed impressive response times of 0.9 s, 1.65 s and 1.8 s, respectively, which was comparable with the FID response. These results suggest that the temporal broadening that we observed is owing to the retentive effect of the GC column, and the intrinsic speed of the graphene heterodyne detector is better than 0.1 s, limited by the rise time of the lock-in amplifier. 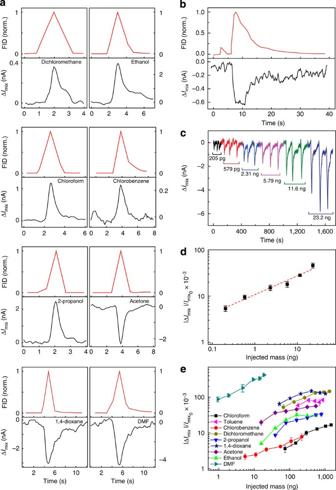Figure 2: Graphene sensor response to different chemical vapours. (a) Comparison of the temporal response of the FID (red) and a graphene sensor (black) to the same injected mass of eight analytes (dichloromethane—66.5 ng, ethanol—78.8 ng, chloroform—296 ng, chlorobenzene—5.5 ng, 2-propanol—78.5 ng, acetone—15 ng, 1,4-dioxane—51.5 ng andN,N-dimethylformamide (DMF)—4.72 ng). The first six analytes were measured on a device withL=7 μm,W=2 μm, at. 1,4-dioxane and DMF were measured on a device withL=9 μm,W=2 μm, at. (b) Temporal response of the FID (red) and a graphene sensor (black) to 205 pg injected mass of DMMP. (c) Chromatographic response of the sensor shown inFig. 2b, to repeated pulses of DMMP at varying mass injections noted in the figure. (d) Measured relative mixing current change of the graphene sensor to DMMP mass injections fromFig. 2c. Linear fit (red-dashed line) to the log–log plot gives a slope of 0.4. (e) Measured relative mixing current response at varying mass injections for nine different analytes. Error bars indandeshow the s.d., over three runs. Analytes were delivered using a 70-cm long guard column at a carrier gas (helium) flow rate of 8 ml min−1. All measurements were carried out in air, at atmospheric pressure and room temperature. Figure 2: Graphene sensor response to different chemical vapours. ( a ) Comparison of the temporal response of the FID (red) and a graphene sensor (black) to the same injected mass of eight analytes (dichloromethane—66.5 ng, ethanol—78.8 ng, chloroform—296 ng, chlorobenzene—5.5 ng, 2-propanol—78.5 ng, acetone—15 ng, 1,4-dioxane—51.5 ng and N , N -dimethylformamide (DMF)—4.72 ng). The first six analytes were measured on a device with L =7 μm, W =2 μm, at . 1,4-dioxane and DMF were measured on a device with L =9 μm, W =2 μm, at . ( b ) Temporal response of the FID (red) and a graphene sensor (black) to 205 pg injected mass of DMMP. ( c ) Chromatographic response of the sensor shown in Fig. 2b , to repeated pulses of DMMP at varying mass injections noted in the figure. ( d ) Measured relative mixing current change of the graphene sensor to DMMP mass injections from Fig. 2c . Linear fit (red-dashed line) to the log–log plot gives a slope of 0.4. ( e ) Measured relative mixing current response at varying mass injections for nine different analytes. Error bars in d and e show the s.d., over three runs. Analytes were delivered using a 70-cm long guard column at a carrier gas (helium) flow rate of 8 ml min −1 . All measurements were carried out in air, at atmospheric pressure and room temperature. Full size image Vapours of a higher boiling point tend to condense more on a surface and thus have longer desorption time. They can be used as a model system to ultimately test the sensor response time and sensitivity. Figure 2b presents the temporal response of the graphene sensor to 205 pg injection of DMMP (boiling point=181 °C) along with the corresponding FID response time. We observed comparable response time for graphene sensor ( t 1/2 =6.1 s) and FID ( t 1/2 =5.5 s). However, DMMP desorption time for graphene sensor (response peak to 90% recovery time, t peak-90%= 28 s) was approximately two times that of FID ( t peak-90%= 13.2 s), indicative of the slow desorption process of DMMP molecules from the graphene surface. To investigate the sensitivity of the graphene heterodyne sensor, in Fig. 2c we plot the sensor response, Δ I mix , in response to repeated doses of DMMP varying from 205 pg to 23.2 ng. It is clear that sensing signal increases with increasing injected mass of DMMP, and that the response is instantaneous and also completely reversible for all the masses under test. Experimentally, the lowest injected mass was 205 pg, corresponding to a concentration of approximately 43 ppb (see Supplementary Note 2 ). To further estimate the graphene sensor’s detection limit, we plot sensor dosage response in Fig. 2d . The sub-linear response in the log–log scale reflects the transient behaviour of vapour pulses interacting with the graphene sensor and is consistent with what has been observed previously with optical sensors [31] . Using a 3σ noise floor (3σ=0.12 nA, Supplementary Fig. 1 ), the detection limit for DMMP is approximately 3 pg in mass or 0.64 ppb in concentration, which to our knowledge is the lowest for any uncoated, pristine nanoelectronic vapour sensor and similar to the best sensitivities reported on chemically coated nanoelectronic vapour sensors [17] , [19] , [20] , [28] . Our order of magnitude calculation also suggests that the noise floor corresponds to ~\n10 4 molecules on the graphene surface (see Supplementary Notes 3 and 4 ). Our graphene heterodyne sensors are also capable of detecting a wide range of vapour analytes without the need of chemoselective surface coatings. Figure 2e plots the graphene sensor dosage response for additional nine analytes. We observed that all analytes showed linear response on the log–log scale at low concentrations and saturate at higher concentrations. The superior performance of the high-frequency heterodyne detection is further evidenced when we contrast the results in Fig. 2c,e with those in Supplementary Fig. 2 , where, using the conventional DC detection method under the identical GC conditions, the GrFET sensor was much less responsive in both response time and sensitivity. The parameters and the experimental results (such as response time and lowest injected mass and so on) of all 13 analytes used in our work are summarized in Supplementary Table 1 . Sensing mechanism for heterodyne vapour detection It is clear that polar molecules yield a stronger signal, whereas the signal from nonpolar molecules is nearly negligible. This distinct sensor response can be understood by examining in equation (3), which is the molecular dipole-induced charge density modulation on graphene, and is proportional to the molecular dipole moment. To further confirm the dipole-detection-based sensing mechanism, we measured the sensor response to a pair of cis - and trans- isomers, cis - and trans -1,2-dichloroethene, with the same injected mass ( Fig. 3a ). It is clear that the polar cis -1,2-dichloroethene (dipole moment=1.9 D) exhibits a strong sensing signal, while the nonpolar trans -1,2-dichloroethene (dipole moment=0 D) only shows minimal response below the 3σ noise floor. 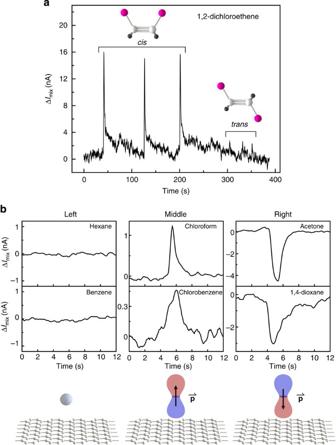Figure 3: Dipole-detection-based sensing mechanism for a graphene heterodyne sensor. (a) Measured mixing current response for a pair ofcis-andtrans-isomers, 1,2-dichloroethene, with the same injected mass of 1.28 μg. Only the polarcis-1,2-dichloroethene shows strong sensor response. The analytes were measured on a device withL=1 μm,W=1 μm, at. (b) Graphene sensor response and the corresponding illustration of the orientation of vapour molecules. Left panel—(top) measured mixing current response for hexane and benzene with an injected mass of 131 and 43.8 ng, respectively. (Bottom) schematic illustration of an analyte with zero dipole moment on graphene. Middle panel—(top) measured mixing current response for chloroform and chlorobenzene with an injected mass of 296 and 55 ng, respectively. (Bottom) schematic illustration of an analyte on graphene with the electronegative cloud (blue) closer to the graphene surface. Right panel—(top) measured mixing current response for acetone and 1,4-dioxane with an injected mass of 156 and 51.5 ng, respectively. (Bottom) schematic illustration of an analyte on graphene with the electropositive cloud (red) closer to the graphene surface.is the molecular dipole moment vector. The analytes were measured on a device withL=7 μm,W=2 μm, at. Figure 3: Dipole-detection-based sensing mechanism for a graphene heterodyne sensor. ( a ) Measured mixing current response for a pair of cis- and trans- isomers, 1,2-dichloroethene, with the same injected mass of 1.28 μg. Only the polar cis -1,2-dichloroethene shows strong sensor response. The analytes were measured on a device with L =1 μm, W =1 μm, at . ( b ) Graphene sensor response and the corresponding illustration of the orientation of vapour molecules. Left panel—(top) measured mixing current response for hexane and benzene with an injected mass of 131 and 43.8 ng, respectively. (Bottom) schematic illustration of an analyte with zero dipole moment on graphene. Middle panel—(top) measured mixing current response for chloroform and chlorobenzene with an injected mass of 296 and 55 ng, respectively. (Bottom) schematic illustration of an analyte on graphene with the electronegative cloud (blue) closer to the graphene surface. Right panel—(top) measured mixing current response for acetone and 1,4-dioxane with an injected mass of 156 and 51.5 ng, respectively. (Bottom) schematic illustration of an analyte on graphene with the electropositive cloud (red) closer to the graphene surface. is the molecular dipole moment vector. The analytes were measured on a device with L =7 μm, W =2 μm, at . Full size image The graphene heterodyne sensor further exhibits strong bi-polar behaviour, as exemplified in Fig. 3b , where the sensor response can be categorized into three types—zero (left panel), positive (middle panel) and negative (right panel). This characteristic can again be traced to the fact that our sensor is responsive to the dipole moment of the surface-adsorbed molecule. Consequently, nonpolar molecules, such as hexane and benzene, show no sensing signal. On the other hand, for polar molecules adsorbed on top of graphene, opposite dipole orientation can lead to opposite signs in the mixing current signal. This bi-polar response of the graphene heterodyne sensor not only adds an additional degree of selectivity for vapour identification, but also hints at its potential as an excellent test bed for elucidating the fundamental molecule–graphene interaction. Graphene heterodyne sensor used in GC chromatograms Rapid separation and detection of chemical vapours are of critical importance for on-site vapour monitoring with portable micro-GC systems. To this end, we present in Fig. 4 the response of the graphene heterodyne sensor (lower panel) and FID (upper panel) to a mixture of eight analytes. The analytes were separated using a combination of GC columns and delivered simultaneously to the graphene sensor and FID using a Y-split ( Fig. 1a ). We observed that the graphene sensor not only responds instantaneously to all polar molecules in the same temporal window as the FID, but also switches sign rapidly for electronegative and electropositive species (relative to graphene) eluted one after the other (6—dioxane and 7—toluene in Fig. 4 ). Pentane and benzene, being nonpolar, were not detected by the graphene sensor. Overall, our proof-of-concept graphene nanoelectronic heterodyne sensor successfully detected all six polar analytes in the mixture with comparable performance as a commercial FID detector. Superior to the bulky destructive FID detector, our graphene sensor is non-destructive, highly compact, and can be readily integrated on-chip with a micro-GC column and read-out circuitry, with zero-dead volume. We also notice the different signs of Δ I mix for 2-propanol in Fig. 2a and Fig. 4 , although all devices processed (including thermal oxide growth) in one batch show consistent behaviour. We attribute this to a substrate effect [32] where end terminations may preferentially orient the molecules through hydrogen bonding, but further detailed investigation is needed. 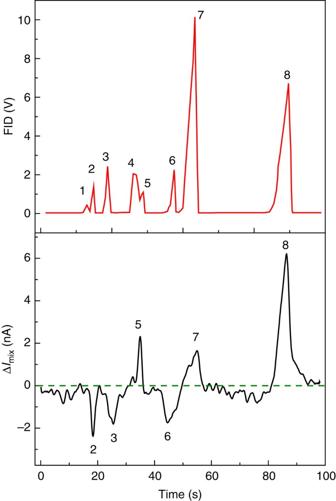Figure 4: GC chromatograms for rapid detection of polar vapour analytes. GC chromatograms obtained simultaneously from the FID (red) and the graphene sensor (black) are shown for a mixture of eight analytes. The mixing current baseline for the graphene sensor is marked by the green-dashed line. Graphene sensor device (L=2 μm andW=2 μm) was operated at. Peaks correspond to: (1)—pentane, (2)—acetone, (3)—2-propanol, (4)—benzene, (5)—chloroform, (6)—1,4-dioxane, (7)—toluene and (8)—chlorobenzene. Analytes were separated and delivered using a combination of a 7.2-m long CP-SIL-5-CB column, a 2.8-m long Carbowax column and a 70-cm long guard column. A Y-split was used for simultaneous delivery of analytes to the FID and the graphene sensor. Figure 4: GC chromatograms for rapid detection of polar vapour analytes. GC chromatograms obtained simultaneously from the FID (red) and the graphene sensor (black) are shown for a mixture of eight analytes. The mixing current baseline for the graphene sensor is marked by the green-dashed line. Graphene sensor device ( L =2 μm and W =2 μm) was operated at . Peaks correspond to: (1)—pentane, (2)—acetone, (3)—2-propanol, (4)—benzene, (5)—chloroform, (6)—1,4-dioxane, (7)—toluene and (8)—chlorobenzene. Analytes were separated and delivered using a combination of a 7.2-m long CP-SIL-5-CB column, a 2.8-m long Carbowax column and a 70-cm long guard column. A Y-split was used for simultaneous delivery of analytes to the FID and the graphene sensor. Full size image Compared with existing nanoelectronic vapour sensor technologies, our graphene nanoelectronic heterodyne sensor presents a number of distinct advantages. First, it is a dipole-detection-based technique, and does not involve the slow dynamics of interface states and charge-transfer processes. Therefore, the sensing response time can be tremendously improved. Second, unlike impedance sensing-based chemicapacitors, the high carrier mobility of graphene transistor provides in situ intrinsic gain for signal amplification (equation 3). Third, graphene can be synthesized in wafer scale and is fully compatible with existing top–down fabrication technology and on-chip electronic circuitry, making graphene nanoelectronic sensors uniquely suited for practical applications. Fourth, the detection limit of graphene heterodyne sensor can be readily pushed down to <100 molecules by device optimization (see Supplementary Note 4 ), opening a door for fundamental studies of molecule–nanomaterial interaction with unprecedented precision. Finally, our heterodyne-sensing technique can be adopted in other types of nanomaterial systems, such as in carbon nanotube and semiconductor nanowire-based sensors, thus having the potential to revolutionize electronic sensor technology as a whole. Fabrication and characterizations of GrFET The graphene FETs were fabricated on a silicon substrate with thermal oxide [30] . A single-layer graphene film was first grown on copper foils using the chemical vapour deposition method. After growth, 950 PMMA (poly(methyl methacrylate)) A2 (Microchem) was spin-coated on one side of the copper substrate and baked at 180 °C for 1 min. Graphene on the uncoated side was removed by 25 s of O 2 plasma etch and then the sample was placed in 0.1 M ammonium persulfate (Sigma-Aldrich) overnight to etch away the copper. Next, the PMMA-coated graphene was transferred from solution onto a thermal oxide substrate and allowed to dry for a day. The PMMA was removed by placing the die in acetone and then isopropyl alcohol (IPA) for 15 min each. Through photolithography, metal deposition and bilayer lift-off processes using LOR 3A (Microchem) and SPR 220-3.0 (Shipley), 0.5 nm titanium/100 nm gold source-drain electrodes were patterned. The graphene channel was patterned using photolithography and 25 s of O 2 plasma etch. A typical device has a graphene channel width of 1–4 μm, and length of 1–9 μm. The graphene devices were first characterized by DC electrical transport measurements before sensing experiments. The I–V g transfer curve for device with channel length, L =7 μm and width, W =2 μm is shown in Supplementary Fig. 3 . The graphene channel was p-doped with a hole carrier mobility of~\n900 cm 2 V −1 s −1 . During all vapour sensing experiments carried out in this work, we kept the gate voltage at 0 V. Graphene heterodyne-sensing measurement scheme For heterodyne sensing, we implemented the graphene transistor as a single-source high-frequency mixer [9] ( Fig. 1a ). An AC-drive voltage, , with a typical amplitude of and frequency of 100 kHz, was provided by a HP 8648B signal generator (Santa Clara, CA, USA). is then amplitude modulated at using the reference signal from a SR830 lock-in amplifier (Stanford Research Systems, Sunnyvale, CA, USA), before it was delivered to the source terminal of the GrFET via a bias tee. The DC bias voltage and DC gate voltage were both maintained at 0 V throughout the sensing measurement. The mixing current was measured at ω m /2 π using the lock-in amplifier, and used as the sensing signal in response to the vapour analytes. Integration of graphene sensor with GC setup The graphene sensor die was capped with a silicon flow channel with 400 μm deep by 400 μm wide, fabricated by a deep reactive ion etch of a patterned silicon wafer for 30 min. The flow channel was carefully aligned to the centre of the die to ensure all the graphene sensors were exposed to the vapour flow ( Fig. 1c ). To secure the flow channel, a small amount of epoxy glue (Norland optical adhesive 81) was used at the edges. Connection of the graphene sensor module to a GC system was achieved by using a 70-cm long guard column (part no. 10029, inner diameter 250 μm, from Restek, Bellefonte, PA, USA). How to cite this article: Kulkarni, G. S. et al. Graphene nanoelectronic heterodyne sensor for rapid and sensitive vapour detection. Nat. Commun. 5:4376 doi: 10.1038/ncomms5376 (2014).